Collective fluorescence enhancement in nanoparticle clusters Many nanoscale systems are known to emit light intermittently under continuous illumination. In the fluorescence of single semiconductor nanoparticles, the distributions of bright and dark periods ('on' and 'off' times) follow Lévy statistics. Although fluorescence from single-quantum dots and from macroscopic quantum dot ensembles has been studied, there has been little study of fluorescence from small ensembles. Here we show that blinking nanorods (NRs) interact with each other in a cluster, and the interactions affect the blinking statistics. The on-times in the fluorescence of a NR cluster increase dramatically; in a cluster with N NRs, the maximum on-time increases by a factor of N or more compared with the combined signal from N well-separated NRs. Our study emphasizes the use of statistical properties in identifying the collective dynamics. The scaling of this interaction-induced increase of on-times with number of NRs reveals a novel collective effect at the nanoscale. The complexity of a system is often tied to its statistical properties. In correlated electron systems, measurements of the statistics of backscattered current (quantum shot noise) have established the elusive fractional quasiparticle charge [1] , [2] , a result of strong electron interactions in the quantum Hall regime. In chemical systems, complexity of the environment produces the fluorescence intermittency or 'blinking' displayed by many types of single emitters, such as single molecules, green fluorescent proteins, light-harvesting complexes, organic fluorophores and semiconductor nanoparticles [3] , [4] . The fluorescence intensity stochastically changes between bright and dark regimes, commonly referred to as on- and off-states. Furthermore, this blinking does not follow a simple two-level quantum jump model, but instead displays approximately power-law (Lévy) statistics over many decades in time [3] , [4] , [5] , [6] , [7] , [8] . Similar non-Poissonian statistics have been observed in electron transport through colloidal nanocrystal (NC) arrays [9] . The origin of the observed Lévy statistics has been investigated extensively, with several models proposed in the 15 years since the first observation of power-law blinking [3] , [4] , [5] . Although the details of the mechanism are still poorly understood, it is thought that NCs become 'dark', cease emitting light, when one of the charge carriers in a photoexcited exciton becomes trapped at the surface of the NC or tunnels off the NC into the environment, leaving a net charge delocalized in the NC core. In the charged core, highly efficient Auger processes lead to rapid nonradiative recombination of subsequent photoexcited excitons. The NC is 'dark' in this 'charge-separated' state; fluorescence resumes once the core regains electrical neutrality [3] , [4] , [5] , [10] , [11] , [12] , [13] , [14] . Recently, the Krauss and Klimov groups observed near-complete suppression of blinking in NCs synthesized with graded shells that greatly reduce the efficiency of Auger recombination, providing strong support for the proposal that dark states involve Auger recombination [10] , [15] . Other mechanisms based on fluctuating nonradiative rates have also been proposed [4] , [16] , [17] . Previous studies [3] , [4] of blinking in NCs focused on single emitters and ensembles of independent emitters. Recently, fluorescence intensity from clusters of close-packed CdSe NCs [18] was found to fluctuate more rapidly than that of isolated NCs, possibly due to interparticle interactions [19] . To determine the number of nanoparticles in a cluster, a high-resolution technique that identifies each CdSe core and its position is required. Our experimental approach ( Fig. 1a ) allows us to directly image both the number of nanoparticles and their location within a cluster, and to measure cluster fluorescence over more than five orders of magnitude in time, from an elementary time step of 0.1 s to several hours. We achieve this by correlating fluorescence microscopy and transmission electron microscopy (TEM) [20] , [21] . 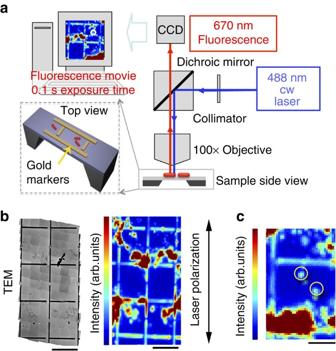Figure 1: Experimental setup and measurement. (a) Schematic of the wide-field fluorescence imaging setup using an upright epi-fluorescence microscope. The sample was illuminated at 488 nm with a continuous-wave solid-state laser. Fluorescence movies (ten frames per s) were captured by a thermoelectrically cooled CCD camera. (b) Fluorescence micrograph of a 18×12 μm2region on the 175×175 μm2Si3N4membrane window (50 nm thickness), and TEM of the same transparent window region patterned with a grid of gold lines, composed by combining 84 high-resolution TEM images. Scale bars, 5 μm. (c) Higher resolution view of a region of fluorescence indicating two blinking clusters (circles) withN=2 and 4. Scale bar, 2 μm. Figure 1: Experimental setup and measurement. ( a ) Schematic of the wide-field fluorescence imaging setup using an upright epi-fluorescence microscope. The sample was illuminated at 488 nm with a continuous-wave solid-state laser. Fluorescence movies (ten frames per s) were captured by a thermoelectrically cooled CCD camera. ( b ) Fluorescence micrograph of a 18×12 μm 2 region on the 175×175 μm 2 Si 3 N 4 membrane window (50 nm thickness), and TEM of the same transparent window region patterned with a grid of gold lines, composed by combining 84 high-resolution TEM images. Scale bars, 5 μm. ( c ) Higher resolution view of a region of fluorescence indicating two blinking clusters (circles) with N =2 and 4. Scale bar, 2 μm. Full size image Previous studies of blinking dynamics in a broad range of nanoscale systems, including individual NCs and nanorods (NRs) [3] , [4] , [5] , [6] , [7] , [8] , showed that most such systems obey power-law or modified power-law dynamics. Specifically, in NCs and NRs, the probability density function (PDF) of on-times follows a truncated power law as a function of on-time, t on [6] , [22] , [23] , where 1< α on <2 is the power-law exponent. The time, τ c,on , is the truncation time, that is, the crossover time between two regimes: the power law at short times and the exponential at long times. At low excitation rates, single NCs typically display τ c,on >10 s, while for single NRs, τ c,on is in the range of 1–10 s, with larger aspect ratio NRs giving smaller τ c,on [6] . Increasing the excitation power decreases τ c,on [13] , [14] , [23] . The PDF of off-times similarly follows a truncated power law with the corresponding power-law exponent α off ~1.3 and the truncation time τ c,off ~1,000 s in NRs [20] . In this article, we investigate blinking in small clusters of semiconductor colloidal NRs comprised of known numbers of particles, N . The cluster fluorescence exhibits collective behaviour: we observe roughly N -fold enhancement of the durations of bright periods ('on-times'), compared with combined fluorescence durations from N separate NRs. We do not, however, observe any change in the durations of off-times. This observed effect of interactions can be figuratively described as a 'campfire effect': although clustering particles together does not help to start the 'fire,' that is, off-times in a cluster are indistinguishable from those for the same number of independent NRs, grouping particles in a cluster does extend the 'burning,' that is, the on-times are strongly increased. Enhancement of on-times in fluorescence from nanoparticle clusters We report analysis of fluorescence intensity versus time, I ( t ), from NR clusters containing N =1 to ~100 nanoparticles ( N for each fluorescence source is determined by TEM imaging), as illustrated in Figure 1b . Figure 1c shows a small region of the fluorescence image at higher resolution, indicating two optically resolvable clusters with N =2 and 4 that were analysed; details of fluorescence data analysis are provided in Methods. We used NRs for this correlation study rather than spherical NCs partly because the elongated NR shape makes it easier to unambiguously distinguish isolated NRs from the background features of the substrate in TEM images ( Fig. 2 ). In addition, compared with spherical NCs with the same emission wavelength, NRs have a greater volume and, hence, greater absorption cross-section than NCs, and are more robust against photobleaching. We used trioctylphosphine oxide (TOPO)-capped CdSe/ZnSe/ZnS core/double shell semiconductor NRs, with a 5.8 nm wide×34 nm long optically active CdSe core and an overall size of 8×38 nm 2 (details of synthesis and characterization given in Methods, Supplementary Methods and Supplementary Fig. S1 ). 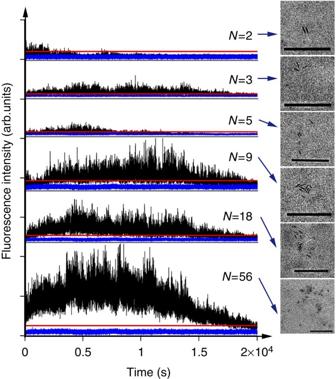Figure 2: Fluorescence of clusters correlated with the number of particles. Fluorescence intensities,I(t), and the corresponding TEM images, in the order of increasing particle number,N=2, 3, 5, 9, 18, 56, background signals (blue curves) and threshold levels (red lines), recorded over 6 h. The scale bars on all TEM images are 200 nm. Figure 2: Fluorescence of clusters correlated with the number of particles. Fluorescence intensities, I (t), and the corresponding TEM images, in the order of increasing particle number, N =2, 3, 5, 9, 18, 56, background signals (blue curves) and threshold levels (red lines), recorded over 6 h. The scale bars on all TEM images are 200 nm. Full size image We determine the blinking statistics of NR clusters from the raw fluorescence time traces ( Fig. 2 ) by setting a threshold distinguishing the fluorescence intensity as 'on' or 'off,' digitizing the trace according to that threshold, and then converting the digitized trace to sequences of 'on' and 'off' times [6] , [20] . We identify the threshold above which a fluorescence signal is considered 'on' using the mean, m dark , and standard deviation, σ dark , of the background intensity measured from a nearby bare region of the substrate. 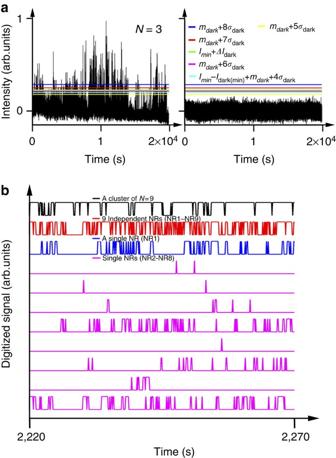Figure 3: Role of interactions in blinking time traces. (a) Fluorescence intensity versus time,I(t), after background subtraction from a cluster withN=3 and its nearby dark region. Different lines (colour) are the different thresholds defined asmdark+8σdark,mdark+7σdark,Imin+ΔIdark,mdark+6σdark,Imin−Idark(min)+mdark+4σdark, andmdark+5σdarkfrom high to low, wheremdark,σdark, ΔIdarkandIdark(min)are the mean, standard deviation, width and the minimum value of the background trajectory, andIminis the minimum value of the trajectory of the cluster. (b) Digitized segment of the fluorescence time trace from a cluster of nine NRs (black), fromN=9 uncorrelated NRs (red) and from a single NR (blue). The red trace is the digitized summation of the digitized traces of nine independent NRs (the one blue trace and eight pink traces) in the experiment. Fluorescence traces for one cluster with N =3 and its nearby substrate region are shown in Figure 3a . We have analysed the trajectories using a range of threshold values (coloured lines in Fig. 3a ). Although it has been shown that blinking statistics are threshold dependent when the threshold is varied significantly [16] , [20] , [24] , our analysis confirms that the trends reported here hold for a wide range of reasonable thresholds (see detailed analysis of on-times for different thresholds in Methods). All results reported in the main paper were determined using a threshold of m dark +7 σ dark (red line in Fig. 3a ) chosen to lie above the background signal from the bare substrate. Figure 3: Role of interactions in blinking time traces. ( a ) Fluorescence intensity versus time, I (t), after background subtraction from a cluster with N =3 and its nearby dark region. Different lines (colour) are the different thresholds defined as m dark +8 σ dark , m dark +7 σ dark , I min +Δ I dark , m dark +6 σ dark , I min − I dark(min) + m dark +4 σ dark , and m dark +5 σ dark from high to low, where m dark , σ dark , Δ I dark and I dark(min) are the mean, standard deviation, width and the minimum value of the background trajectory, and I min is the minimum value of the trajectory of the cluster. ( b ) Digitized segment of the fluorescence time trace from a cluster of nine NRs (black), from N= 9 uncorrelated NRs (red) and from a single NR (blue). The red trace is the digitized summation of the digitized traces of nine independent NRs (the one blue trace and eight pink traces) in the experiment. Full size image Just from inspecting excerpts of the digitized time traces (one example for N =9 is given in Fig. 3b ), it is evident that the clusters exhibit much longer on-times than a combined signal from the same number of separate NRs measured from the same chip. The increased on-times are also clearly manifested in the shape of the on-time PDF that extends to longer on-times ( Fig. 4a ). 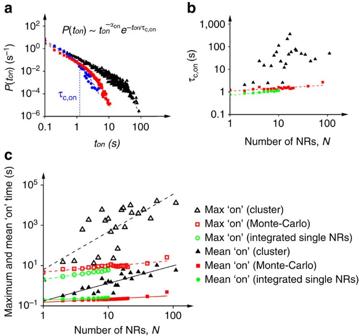Figure 4: Role of interactions in blinking statistics. (a) Probability density of on-times from the traces shown inFigure 3b. The effects of interactions are seen as a cutoff timeτc,onin the Lévy distribution of a cluster (black) compared with the correspondingτc,onfor integrated signals of nine independent particles (red) and for a single NR (blue). (b) Scaling ofτc,onwith the cluster sizeN(black triangles) compared with that ofNisolated NRs located on the same chip (green squares) and with results from a Monte-Carlo simulation ofNnon-interacting particles (red squares). (c) Scaling of mean and maximum on-times with the cluster sizeN(open and solid black triangles, respectively) compared with on-times obtained from integrating signals fromNisolated NRs located on the same chip (open and solid green circles) and with results from a Monte-Carlo simulation ofNnon-interacting particles (open and solid red squares). The Monte-Carlo simulated mean and maximum on-times (red) qualitatively agree with corresponding measured mean and maximum on-times from a collection of non-interacting NRs (green). Although there is some variability of the PDF parameters of the measured individual NRs, the Monte-Carlo simulations assume identicalτc,on(off)andαon(off)for all NRs. Figure 4: Role of interactions in blinking statistics. ( a ) Probability density of on-times from the traces shown in Figure 3b . The effects of interactions are seen as a cutoff time τ c,on in the Lévy distribution of a cluster (black) compared with the corresponding τ c,on for integrated signals of nine independent particles (red) and for a single NR (blue). ( b ) Scaling of τ c,on with the cluster size N (black triangles) compared with that of N isolated NRs located on the same chip (green squares) and with results from a Monte-Carlo simulation of N non-interacting particles (red squares). ( c ) Scaling of mean and maximum on-times with the cluster size N (open and solid black triangles, respectively) compared with on-times obtained from integrating signals from N isolated NRs located on the same chip (open and solid green circles) and with results from a Monte-Carlo simulation of N non-interacting particles (open and solid red squares). The Monte-Carlo simulated mean and maximum on-times (red) qualitatively agree with corresponding measured mean and maximum on-times from a collection of non-interacting NRs (green). Although there is some variability of the PDF parameters of the measured individual NRs, the Monte-Carlo simulations assume identical τ c,on(off) and α on(off) for all NRs. Full size image We quantify the increased on-times by calculating the mean and maximum on-times, as well as by fitting the on-time probability densities to a truncated power law, equation (1) (fitting method described in Supplementary Figure S2 and Supplementary Methods ). We use the fit to the truncated power law simply as a way to characterize the range of observed on-times; it is not clear that cluster fluorescence should be expected to display truncated power-law statistics, and the variation in power law exponents between individual NRs would be expected to affect the distribution obtained from combining independent NRs. From such fits, the truncation time τ c,on can be as much as two orders of magnitude greater for clusters than for the combined signal from the same number of isolated particles ( Fig. 4b ). Figure 4c shows the maximum and mean on-times (open and solid black triangles) for 120 clusters of various sizes; each point in the figure represents the average from all clusters with the same particle number, N . These results are compared with both the signal obtained by combining individual signals from N isolated single particles that were found on the same chip ( Fig. 4c , open and solid green circles) and a Monte-Carlo simulation combining N independent trajectories following truncated power-law blinking dynamics ( Fig. 4c , open and solid red squares). The combined experimental data were averaged over 30 random combinations of single NRs and the Monte-Carlo data were generated independently for each N . Individual signals from N separate NRs were combined either before or after the individual signals were digitized as described in Supplementary Methods ; both approaches, compared in Supplementary Figure S3 , yield the same conclusions. For clusters, we find that both maximum and mean on-times increase by a factor of N or more over the same number of independent NRs (both data and simulated). For example, the maximum on-time of ~10 s for N =10 independent NRs increases to ~1,000 s for clusters of ten NRs. Figure 4c displays the average over all measured clusters of a given N ; in addition, all clusters with N >6 and more than 80% of clusters with 1< N ≤ 6 exhibit enhanced on-times compared with both N measured individual NRs and Monte-Carlo simulations. The cluster data in Figure 4b,c show more scatter than either the combined data from independent NRs or the Monte-Carlo simulation. One likely explanation for some of the scatter is that, for the combined independent NRs and the Monte-Carlo simulation, N is the number of emitting NRs; for the clusters, N is the number of NRs in the cluster counted from the TEM images, and may therefore be greater than the number of emitting NRs in each cluster, because a significant fraction (up to ~50–70%) of NRs may be permanently dark [20] , [21] , [25] . For the clusters, N therefore represents an upper bound on the number of emitting NRs. The enhancement of on-times may therefore be even more dramatic than Figure 4b,c suggests. Another likely source of scatter is the variation in inter-NR distances in a cluster, which is expected to affect the strength of any interaction. As shown in Figure 2 , in some clusters all NRs are closely packed, while in most, some are close-packed and others are more widely separated. Although the distribution of on-times differs dramatically from clusters to combined independent NRs, we see no effect of interactions on the mean or maximum off-times within our experimental resolution ( Fig. 5a ). Furthermore, the total time spent on (obtained by summing all on-times from a given experiment) does not increase by more than one order of magnitude. 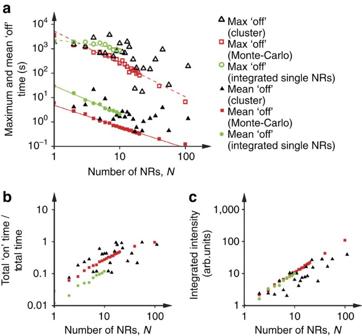Figure 5: Scaling of blinking parameters. (a) Scaling of mean and maximum off-times inversely with the cluster sizeN(open and solid black triangles) compared with off-times obtained from integrating signals fromNisolated NRs found on the same chip (open and solid green circles) and with results from a Monte-Carlo simulation ofNnon-interacting particles (open and solid red squares). (b) Scaling of the fraction of the total time spent in the on-states withN(black triangles) compared with data obtained from integrating signals fromNisolated NRs found on the same chip (green circles), and with results from a Monte-Carlo simulation ofNnon-interacting particles (red squares). (c) Scaling of the integrated intensity withN(black triangles) compared with data obtained from integrating signals fromNisolated NRs found on the same chip (green circles) and with results from a Monte-Carlo simulation ofNnon-interacting particles (red squares). This is shown in Figure 5b (compare green circles and black triangles). This indicates that cluster fluorescence trajectories are composed of fewer on-events that are on average longer, whereas trajectories combined from multiple independent particles are composed of a greater number of shorter on-events ( Supplementary Fig. S4 ). Figure 5: Scaling of blinking parameters. ( a ) Scaling of mean and maximum off-times inversely with the cluster size N (open and solid black triangles) compared with off-times obtained from integrating signals from N isolated NRs found on the same chip (open and solid green circles) and with results from a Monte-Carlo simulation of N non-interacting particles (open and solid red squares). ( b ) Scaling of the fraction of the total time spent in the on-states with N (black triangles) compared with data obtained from integrating signals from N isolated NRs found on the same chip (green circles), and with results from a Monte-Carlo simulation of N non-interacting particles (red squares). ( c ) Scaling of the integrated intensity with N (black triangles) compared with data obtained from integrating signals from N isolated NRs found on the same chip (green circles) and with results from a Monte-Carlo simulation of N non-interacting particles (red squares). Full size image Figure 5c shows that the total integrated intensity, I int , of clusters increases sublinearly with the number of NRs, although the decrease compared with the independent combined NRs is not dramatic. (The total integrated intensity is calculated as I int = ∑ i =1 I int / M , with I i the background-subtracted intensity for the i th time interval of 0.1 s from a particular time trace.) One possible explanation for the sublinearity is that the number of optically active NRs in the cluster is consistently less than N . This is plausible, because, as previously discussed, not all NRs observed by TEM are necessarily emitting [25] . Another possibility is that interactions between the NRs in closest proximity significantly reduce simultaneous emission from multiple NRs within the cluster. Others have previously established that individual NCs are single-photon emitters [26] , [27] , [28] . In the future, submicrosecond autocorrelation function (ACFs) measurements of cluster emission, to correlate particle number with the degree of photon antibunching, may clarify further under what circumstances multiple particles within clusters emit independently. Scaling of on- and off-times with particle number We now consider the theoretical scaling of the mean and maximum on- and off-times with the cluster size N . To get an idea of how the mean and maximum on- and off-times should scale in the absence of interactions, first let us understand what would happen in the simplest case where each nanoparticle blinking is governed by Poissonian distributions of on- and off-times, assuming the ratio r = t off / t on ≫ 1 ( r approaches 150 from Figs 4c and 5a for N =1). For large r , the intensity trajectory is a sequence of bright spikes separated by long dark intervals; both mean and maximum duration off-intervals would be of the order t off . Adding N such uncorrelated signals will increase the rate of the spikes N -fold, thereby reducing both the mean and maximum off-times by a factor of N , while negligibly affecting the mean and maximum duration of the on-spikes, as long as N < r . (If N ~ r , the overlap of the on-spikes will become significant and both the mean and maximum values of the on-times will start increasing with N .) This argument applies qualitatively to truncated power-law statistics as well, as long as the cutoffs for on- and off-distributions are much shorter than the observation time, as is the case in our measurements. Monte-Carlo simulations for summing either Poissonian or truncated Lévy uncorrelated distributions support these observations. Figure 4c (open and solid red squares) shows the Monte-Carlo simulations of the maximum and mean on-times for N independent particles with the same fluorescence statistics, assuming the same range of power-law exponents α on , α off and truncation times (see equation (1) and Supplementary Methods ). The statistical parameters acquired from the Monte-Carlo simulated signal qualitatively agree with those acquired from the signal from a collection of non-interacting NRs. The quantitative discrepancies are attributed to the variability of the PDF parameters of the individual NRs, whereas the Monte-Carlo simulations are performed using identical τ c,on(off) and α on(off) for all NRs. From Figure 5a , we see that, in agreement with the above reasoning, both mean and maximum off-times for N non-interacting particles indeed decay approximately as 1/ N . This property persists also for the clusters, at least within our experimental errors. For the on-times ( Fig. 4c ), the difference from the uncorrelated picture is profound: both mean and maximum on-times grow very rapidly with N even at N ~1, while the off/on ratio r ~150. In contrast, the same quantities for the non-interacting particles change very little with N . The parameters of the on-time statistics for a cluster and for N non-interacting particles differ approximately by a factor of ~N 1.6 for maximum on-times and by a factor of ~ N 0.7 for mean on-times. This significant scaling of the statistics of on-times with N reveals the extensive character of the observed effect, and implies that the novel behaviour is indeed collective. Autocorrelation function analysis We also examine ACFs of fluorescence trajectories of individual NRs and clusters ( Fig. 6a ). We define the ACF as where I ( t ) is the fluorescence intensity at time t , averages are performed over all t , and τ is the lag time. 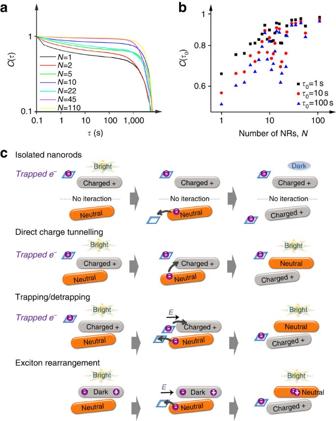Figure 6: Autocorrelation functions and schematic of possible charging processes. (a) Autocorrelation functions of individual NRs (black curve) and NR clusters ofN=2, 5, 10, 22, 45, 110 (shown in colour). (b) Scaling of the values of autocorrelation functions atτ0=1, 10 and 100 s with the cluster sizeN. (c) Possible charging processes in two isolated NRs and in an interacting cluster ofN=2 NRs, showing how interactions can keep the NR cluster bright. In all cases, one rod is initially charged and the other neutral, so initially one rod in the pair is bright. In the two isolated rods, when charge tunnelling causes the neutral rod to become charged and thus dark, the pair also becomes dark. In the interacting cluster, when the neutral rod becomes charged, the three different types of interactions (described in the text) can each cause the other, charged rod to become neutral simultaneously, keeping the pair bright. In the diagram of exciton rearrangement, the electric field is the net field along the direction of the separation of the charges. The ACFs shown in Figure 6a are the average over the ACFs of clusters with the same particle number, N . At shorter lag times ( τ <100 s), C ( τ ) decays faster for individual NRs (black curve) and its decay slows as N increases (colour). Figure 6b shows the average ACF values for all clusters studied as a function of N , at fixed lag times, τ 0 =1, 10 and 100 s; C ( τ 0 ) increases with N for all τ 0 . This means that the fluorescence trajectory of a cluster correlates with itself over longer times in larger clusters, consistent with our observation of the strong increase of on-times ( Fig. 4c ). Finally, we note that the ACF analysis of NC clusters reported in refs 18 and 29 found that instead, the ACF decays faster for clusters than for individual NCs. The difference may be due to the use of spherical NCs rather than NRs in refs 18 and 29 , and the different sample preparation method used, resulting in clusters with differing degrees of packing. As that work did not address differences in the blinking parameters, we cannot compare findings of the particle number dependence of on- and off-times. Figure 6: Autocorrelation functions and schematic of possible charging processes. ( a ) Autocorrelation functions of individual NRs (black curve) and NR clusters of N= 2, 5, 10, 22, 45, 110 (shown in colour). ( b ) Scaling of the values of autocorrelation functions at τ 0 =1, 10 and 100 s with the cluster size N . ( c ) Possible charging processes in two isolated NRs and in an interacting cluster of N= 2 NRs, showing how interactions can keep the NR cluster bright. In all cases, one rod is initially charged and the other neutral, so initially one rod in the pair is bright. In the two isolated rods, when charge tunnelling causes the neutral rod to become charged and thus dark, the pair also becomes dark. In the interacting cluster, when the neutral rod becomes charged, the three different types of interactions (described in the text) can each cause the other, charged rod to become neutral simultaneously, keeping the pair bright. In the diagram of exciton rearrangement, the electric field is the net field along the direction of the separation of the charges. Full size image To reconcile the dramatic enhancement of maximum and mean on-times with the unchanged off-time distribution for the cluster, and drawing on the Auger recombination model for blinking [3] , [4] , [5] , [10] , [11] , [12] , [13] , [14] we propose two kinds of possible in-cluster charging processes, each one potentially capable of keeping at least one NR uncharged and, hence, bright: direct charge tunnelling between closely located NRs, and electric field-mediated charge redistribution, which can either be static (involving exciton rearrangement) or dynamic (involving coordinated trapping and detrapping). For the smallest possible cluster ( N= 2), Figure 6c shows a schematic diagram of each of these processes, compared with the charge states of two independent NRs.For two NRs, there are three possible charge state combinations: neutral–neutral, charged–neutral and charged–charged (the latter one being dark). Here the charged state corresponds to an electron trapped in the NR shell or in the local environment, with the hole left on the NR rendering it dark [3] , [4] , [5] , [10] , [11] , [12] , [13] , [14] . The charged–neutral state can become dark if an electron from the neutral NR also becomes trapped, causing it to switch off. In a cluster, this electron may instead recombine with the hole in the neighbouring dark NR, rendering the latter neutral (direct charge tunnelling, shown in Fig. 6c ). Alternatively, when the electron from the neutral NR is trapped, the resulting electric field change may cause the previously dark NR to switch on without direct charge transfer between the NRs. This may happen either dynamically, by provoking recombination of the adjacent trapped electron with its dark NR core (coordinated trapping and detrapping, shown in Fig. 6c ), or statically, by the field change reducing the overall static field acting on the exciton in the dark NR (exciton rearrangement, shown in Fig. 6c ). Indeed, it has been shown experimentally [30] that a NR can be switched 'off' or 'on' by a static field, which increases or decreases, respectively, the spatial electron-hole separation. Such a field in the dark NR may originate either from the residual crystal field in a NR [30] or due to charges in the environment. Estimates of the field strengths involved in the field-mediated processes are provided in Supplementary Note 1 . Either of the suggested charge movements would facilitate combining the on-times of individual NRs in a continuous sequence, in a cluster of any size, as long as at least one NR remains bright. Although the total time spent in the on state should increase under either of these scenarios, the observed increase ( Fig. 5b ) of the fraction of time spent in the on state grows relatively slowly with N . This is expected near saturation, when this fraction approaches unity, resulting in the large clusters emitting most of the time. Notably, all of the suggested mechanisms would keep the distribution of off-times unchanged from what would be expected for independent NRs, in agreement with our observations. This is because an off-time for either the cluster or the combined independent NRs corresponds to a time during which there is no charge transfer into or out of any of the individual NRs. Estimates of the distance ranges of these charging processes show that all are strongly sensitive to the edge-to-edge separation between NRs, and thus the dominant interactions should occur between the closest NRs in clusters. Direct tunnelling is only likely between close-packed NRs separated by 1–2 nm. For spherical core-shell NCs, Kuno et al . [12] estimate that the range of experimentally observable blinking rates (from 10 kHz to 0.01 Hz) could correspond to tunnelling between the core and trap sites on the substrate 1–2 nm away from the surface of the NC shell. This suggests direct charge tunnelling between close-packed NRs in our clusters is plausible. Furthermore, tunnelling could involve an intermediate state on the silicon nitride substrate between the NRs, as long as its lifetime is sufficiently short that the complete charge transfer process occurs in less than our temporal resolution of 0.1 s. This could potentially extend the distance range somewhat. The dynamical effect of coordinated trapping and detrapping depends on the details of the trapping potential. Our estimates ( Supplementary Note 1 ) suggest that it is also most effective between NRs separated by just a few nm, because this charge rearrangement produces an effective dipole field that decays over relatively short distances. Finally, static exciton rearrangement may act on distances up to 8–10 nm ( Supplementary Note 1 ) for NRs suitably aligned with the field of the trapped charge, so it may act on somewhat longer distances than the other mechanisms. All of the above interaction mechanisms based on charge processes are consistent with the geometry of our clusters. Analysis of TEM images of the clusters shows that ~85% of the clusters in our study include at least two NRs separated by 2 nm or less from edge to edge, and that larger clusters have greater percentages of NRs next to each other. However, almost none of the N >2 clusters are fully close-packed; most clusters have between 50 and 80% of NRs with at least one neighbour within 2 nm or less. (Details are provided in Supplementary Note 1 , Supplementary Figs S5 and S6 .) Supplementary Table S1 shows the fraction of close-packed NRs in 74 clusters with N =2–110. The complexity of the observed statistics most likely reflects the presence of more than one mechanism at work, and possibly all of them. Indeed, although many of the proposed models for blinking are based on charging processes, an alternative class of models based on fluctuating nonradiative rates [16] , [17] , [31] , [32] has also been proposed. In these models, blinking is associated with opening and closing certain nonradiative exciton recombination pathways involving localized surface states. With such a mechanism, resonant energy transfer, resulting in exciton transfer between NRs in a cluster, would be likely to affect the blinking statistics significantly, potentially by transferring excitations from dark NRs to bright ones, although it is not immediately clear to us how energy transfer within such a mechanism could produce our observed sequencing of on-states while leaving the off-statistics unchanged. Regardless of the still debated blinking framework, the apparent interaction effect observed here should introduce constraints and couplings between the single-NR parameters of these and other possible models of blinking, and could help either validate them or rule them out. Such investigation is beyond the scope of this work. To further test the mechanism behind the observed enhancement, we analysed the mean and maximum on-times versus mean interparticle separations (the simplest case of N =2 is shown in Supplementary Fig. S7 ). We find that the on-times are too scattered to observe any clear trend with interparticle separations. This scatter can result from a large variation in blinking parameters of the individual NRs that comprise the clusters so that no clear trends are observable when measuring ensembles of clusters with fixed N . Another potentially important factor is the uncertainty in the actual number of emitting NRs within particular clusters. For example, a pair of NRs observed in TEM imaging may include only a single emitting NR. To eliminate the confounding effects of ensemble averaging, we also attempted to guide the NR assembly into ordered clusters by patterning surface features on silicon nitride substrates and by surface modifications, but subsequent TEM imaging revealed that the resulting clusters, though spatially more localized, still contained a large degree of disorder. To unequivocally explain the underlying interaction mechanisms, small NR clusters with well-controlled assembly patterns and interparticle separations are needed. This is a challenging goal for future experiments as reproducible ordered assembly of CdSe nanoparticles is still a difficult task. In conclusion, we observed a collective effect in the fluorescence of disordered nanoparticle clusters resulting in longer bright periods than measured and simulated on collections of independent particles. Although clusters do not emit more intensely, the emission periods are prolonged. One possible explanation for our observations is that particles may alternate with each other in bright and dark states to extend the overall emission period. The long on-times observed here may also explain earlier observations on very large NR ensembles [21] ( N >10,000) where the onset of the power-law decay in ensemble fluorescence occurred much later than predicted by a statistical model based on non-interacting single-particle dynamics [21] , [33] , [34] . Finally, CdSe NRs have promising applications as nanoscale emitters, both as fluorescent labels in applications that do not require ultra-small nanoprobes and as single-photon sources. Our study suggests that small NR clusters may be usable as nanoscale light sources with long emission times. For example, maximum emission times can be extended from 10 to 1,000 s for clusters with ten NRs. The dramatic increase of up to two orders of magnitude in emission times reported here demonstrates that interparticle interactions in clusters can favourably modify blinking dynamics. Sample preparation and experimental procedures Low stress 50-nm-thick silicon nitride (Si 3 N 4 ) membranes [35] were used as substrates, because they are transparent in TEM and show low fluorescence background [36] . Gold markers, to aid in locating the NRs, were fabricated on the membrane by electron beam lithography in the shape of 5×5 μm 2 squares. NR solutions in toluene were deposited onto the substrate by drop-casting (7 μl). The dimensions of the NRs were determined by analysing TEM images of more than 200 NRs using ImageJ software. The core sizes were measured to be 5.8±0.3 nm in diameter and 34±3 nm in length and the core/double shell NRs to be 8±0.7 nm×38±6 nm. Therefore, the double shell of our nanorods is estimated to be 1.1 to at most 2 nm thick, determined from the average diameters and lengths, respectively. The shell is thinner along the length of the nanorods and the greatest thickness is along the ends. Wide-field fluorescence imaging ( Fig. 1a ) was performed at room temperature in air, using an upright epi-fluorescence microscope (Nikon Eclipse 80i, Nikon) with a Nikon Apo 100×0.95 NA dry objective and a 670±25 nm emission filter (Chroma 670/50M, Chroma). To obtain enough clusters of NRs, a fairly high concentration of NRs (~10 nM) was deposited on the substrate, producing many extended regions in which individual clusters were not optically resolvable; we only analysed data from clusters optically resolvable from their neighbours. The sample was illuminated at 488 nm (100 W cm −2 ) with a continuous-wave solid-state laser (Coherent Sapphire, Coherent). Fluorescence movies (ten frames per s, up to ~7 h long) were captured by a thermoelectrically cooled CCD (charge-coupled device) camera (PhotonMAX, Princeton Instruments). The fluorescence intensity of each emitter was determined in each frame throughout the entire movie and it was corrected by subtracting a background from a nearby dark region [20] . The mechanical stability of our setup, with a drift of 100 nm h −1 , allows us to trace the fluorescence dynamics for many hours [20] , [21] . The small mechanical drift was accounted for by offsetting the position of the recorded frames appropriately during data analysis. The analysis of fluorescence statistics, previously described in detail [6] , [20] , is performed after thresholding and subsequent digitizing of a thresholded signal and the conclusions in this paper hold qualitatively for a range of thresholds. Fluorescence data collected from independent measurements on two different chips match very well ( Supplementary Figs S8 and S9 ). Statistical analysis of various temporal sub-segments within the fluorescence movie showed no significant or systematic change in the blinking parameters of single NRs over the duration of the experiment [21] . Still, effects of sample degradation over time can not be excluded. Some clusters become dark over the course of the experiment, in which case the maximum on-times reported in Figure 4c may be smaller than what may be possible otherwise. The digitized trace of nine independent NRs (red) in Figure 3b was the digitized summation of the digitized traces of nine independent NRs (blue and pink traces) in the experiment. Figure 3b shows the overlapping effect when these nine independent traces (blue and pink traces) sum up to produce the red trace. Analysis of correlated TEM and fluorescence data Following fluorescence imaging, we located NRs relative to the nearest gold markers using TEM (JEOL 2010, JEOL). TEM was always performed after the fluorescence measurements to avoid sample contamination and degradation. Approximately 1,000 high-resolution TEM images of 2×1.4 μm 2 areas were collected and then combined together to reconstruct the larger 175×175 μm 2 Si 3 N 4 membrane windows of two chips ( Supplementary Figs S8 and S9 ). TEM image analysis was performed using the Image Processing Toolbox application in Matlab to process data from the whole chip. Image registration was applied to align the fluorescence and TEM images of the same sample area by using the gold grid pattern on the substrate, mapping four points on each image and transforming (for example, rotating or expanding) one image to overlay it on top of the other. The uncertainty in overlaying the two images is <100 nm, which is better than the spatial resolution of resolving two nearby fluorescent sources (~330 nm). The measurement error in the number of NRs, N , comes primarily from TEM imaging and is estimated to be ±1 for N ≤10 and 10% for N >10. The number of emitting NRs may be significantly smaller. Determination of fluorescence intensity versus time from fluorescence movies Fluorescence from a single emitter was determined by integrating the signal from the appropriate 'segment' (region) of a fluorescence image. We determine the segments for individual emitters by correlating them with TEM images ( Fig. 1b ). For the analysis, we chose clusters that can be optically resolved from nearby emitters. The resolution determined by the emission wavelength (λ) and the numerical aperture (NA) of our setup can be calculated as λ/2 NA ~330 nm, which corresponds to ~2 pixels of the magnified image on our CCD detector, so that the fluorescence from an emitter is spread over an area ranging from 2×2 pixels to 4×6 pixels in our samples. The fluorescence intensity of each cluster was determined in each frame throughout the entire movie and it was corrected by subtracting the background measured from a nearby bare region of the substrate; for example, e is the background segment of a and c, and f is the background segment of d ( Fig. 7 ). 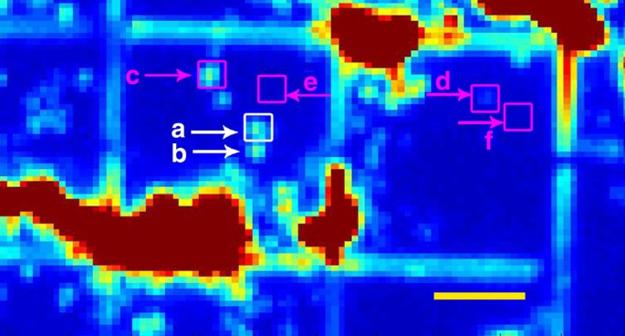Figure 7: Determination of fluorescence segments and its background. Fluorescence micrograph of a 13×9 μm2region on the 175×175 μm2Si3N4membrane window (50 nm thickness).Scale bar, 2 μm. (a, c, d) Three clusters used in the data analysis, withN=2, 4 and 2, respectively. (b) Another cluster near the cluster a. (e) The background segment of clusters a and c. (f) The background segment of cluster d. Figure 7: Determination of fluorescence segments and its background. Fluorescence micrograph of a 13×9 μm 2 region on the 175×175 μm 2 Si 3 N 4 membrane window (50 nm thickness).Scale bar, 2 μm. (a, c, d) Three clusters used in the data analysis, with N =2, 4 and 2, respectively. (b) Another cluster near the cluster a. (e) The background segment of clusters a and c. (f) The background segment of cluster d. Full size image The centres of the fluorescence segments that we analysed are separated by at least 3 pixels from the centres of their nearest neighbours. Segments a, c and d are three emitting spots included in the data analysis with N =2, 4 and 2, respectively, and b is another bright spot near a. However, the brightness spreads out from the centre of some emitters (for example, a and c) to the edges of the neighbouring spots, though the centres (local maximal brightness) of them can be well resolved. To study the effect of possible brightness overlaps, out of the 120 spots on this chip, we then chose a subset of 42 clusters that satisfy a stricter criterion, that is, that have completely isolated bright spots (for example, cluster d) with a dark surrounding region. Supplementary Figure S10 shows the maximum and mean on-times for the 42 isolated clusters (half-solid pink squares and cyan circles). These results are compared with on-times obtained from all 120 bright spots in Figure 4c (open and solid black triangles), the signal obtained by combining individual signals from N separate particles that were found on the same chip ( Fig. 4c , open and solid green circles) and with a Monte-Carlo simulation combining N -independent trajectories ( Fig. 4c , open and solid red squares). The data from the subset of 42 completely isolated bright spots match very well with the data from all 120 spots, which shows that including closely adjacent clusters does not affect the on-times within the experimental resolution. Background correction and definition of threshold Silicon nitride (Si 3 N 4 ) membrane devices show a slight background fluorescence signal that is not homogenous throughout the whole substrate. Consequently, each fluorescent segment was corrected with respect to a dark segment in its vicinity. Moreover, the background can evolve slightly over time for very long fluorescence movies. To account for these changes, we fit the background signal with a fourth-order polynomial that is subtracted from the fluorescence segment (for example, the time trajectory from a cluster with N =3 and a nearby dark region, Supplementary Fig. S11a ). We have analysed the measured time-traces for a range of thresholds as illustrated in Supplementary Figure S11b and for six different threshold levels defined as m dark +8 σ dark , m dark +7 σ dark , I min +Δ I dark , m dark +6 σ dark , I min − I dark(min) + m dark +4 σ dark , and m dark +5 σ dark from high to low, where m dark , σ dark , Δ I dark and I dark(min) are the mean, standard deviation, width and the minimum value of the background trajectory, and I min is the minimum value of the trajectory of the cluster. Although it has been shown that blinking statistics are threshold dependent when the threshold is varied significantly [16] , [20] , [24] , our analysis confirms that the trends reported here hold over the entire threshold range tested, that is, from m dark +5 σ dark up to m dark +8 σ dark , while the absolute on- and off-time durations in the main paper depend on the exact threshold chosen, with higher thresholds yielding effectively shorter on-times ( Fig. 8a ). Another example of a time trajectory after background subtraction from a single NR is shown in Supplementary Figure S12 . The coloured lines are thresholds defined the same way as those in Supplementary Figure S11b and the 'on' times and the truncation time τ c,on are lower with higher thresholds for this single NR ( Fig. 8b ). Changing the threshold within this range does not change on-time versus cluster size N significantly ( Supplementary Fig. S13 ). The time durations and probability densities reported in the main article were determined using a threshold of m dark +7 σ dark , in the middle of this range. 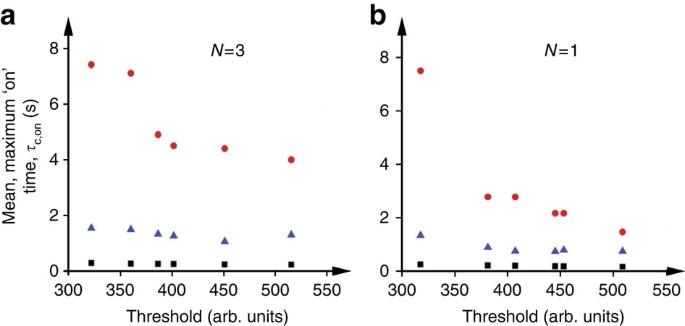Figure 8: Effect of threshold on mean and maximum 'on' times andτc,on. Scaling of mean (black squares), maximum 'on' times (red circles) andτc,on(blue triangles) of a cluster with (a)N=3 and (b)N=1. The thresholds are defined inSupplementary Figures S11 and S12. Figure 8: Effect of threshold on mean and maximum 'on' times and τ c,on . Scaling of mean (black squares), maximum 'on' times (red circles) and τ c,on (blue triangles) of a cluster with ( a ) N =3 and ( b ) N =1. The thresholds are defined in Supplementary Figures S11 and S12 . Full size image Blinking time distributions for single nanoparticles have also been shown to depend on the time resolution of the intensity–time trace [24] . However, in this work, we compare measurements and simulations all made with the same time resolution. Consequently, although the specific values of the maximum and average on and off times, and the truncation time, would be expected to change with time resolution, the choice of time resolution should affect all the data the same way and thus not affect the comparisons. How to cite this article: Wang, S. et al . Collective fluorescence enhancement in nanoparticle clusters. Nat. Commun. 2:364 doi: 10.1038/ncomms1357 (2011).